Epithelial rotation promotes the global alignment of contractile actin bundles duringDrosophilaegg chamber elongation Tissues use numerous mechanisms to change shape during development. The Drosophila egg chamber is an organ-like structure that elongates to form an elliptical egg. During elongation the follicular epithelial cells undergo a collective migration that causes the egg chamber to rotate within its surrounding basement membrane. Rotation coincides with the formation of a ‘molecular corset’, in which actin bundles in the epithelium and fibrils in the basement membrane are all aligned perpendicular to the elongation axis. Here we show that rotation plays a critical role in building the actin-based component of the corset. Rotation begins shortly after egg chamber formation and requires lamellipodial protrusions at each follicle cell’s leading edge. During early stages, rotation is necessary for tissue-level actin bundle alignment, but it becomes dispensable after the basement membrane is polarized. This work highlights how collective cell migration can be used to build a polarized tissue organization for organ morphogenesis. During development, tissue morphogenesis requires precise coordination of individual cell behaviours and reciprocal interactions between cells and their extracellular matrix. The Drosophila egg chamber provides a highly amenable system to identify molecular mechanisms underlying changes in tissue and organ shape [1] . Egg chambers are multicellular structures within the fly ovary that will each give rise to a single egg. They are composed of a germ cell cluster surrounded by an epithelial layer of follicle cells. The basal surface of the epithelium is in contact with a basement membrane extracellular matrix, which encapsulates the egg chamber ( Fig. 1a,b ). Egg chambers are assembled in an anterior ovarian region known as the germarium and are then organized into a developmental array called an ovariole ( Fig. 1a ). Each egg chamber progresses through 14 developmental stages before forming an egg. 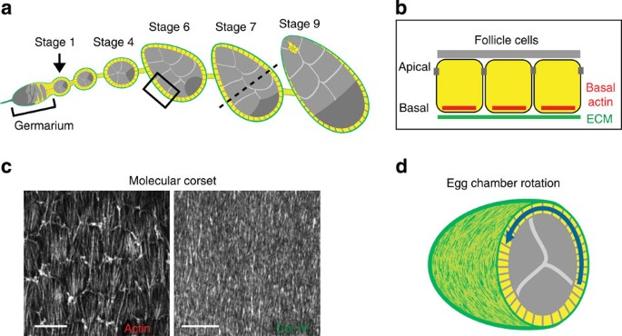Figure 1: Overview of key concepts in egg chamber elongation. (a) Illustration of an ovariole, a developmental array of egg chambers. Egg chambers are spherical when they bud from the germarium and then lengthen along their anterior–posterior axes as they develop. (b) Blowup of the boxed region inahighlighting the apical–basal axis of the follicle cell epithelium. (c) The ‘molecular corset’ consists of parallel arrays of actin bundles at the basal epithelial surface (stage nine) and fibril-like structures in the adjacent basement membrane (stage seven). Laser-scanning confocal images. Scale bar, 10 μm. (d) Transverse section through a stage seven egg chamber, as shown by the dashed line ina. The egg chamber rotates within the surrounding basement membrane (illustration adapted from ref.32). Figure 1: Overview of key concepts in egg chamber elongation. ( a ) Illustration of an ovariole, a developmental array of egg chambers. Egg chambers are spherical when they bud from the germarium and then lengthen along their anterior–posterior axes as they develop. ( b ) Blowup of the boxed region in a highlighting the apical–basal axis of the follicle cell epithelium. ( c ) The ‘molecular corset’ consists of parallel arrays of actin bundles at the basal epithelial surface (stage nine) and fibril-like structures in the adjacent basement membrane (stage seven). Laser-scanning confocal images. Scale bar, 10 μm. ( d ) Transverse section through a stage seven egg chamber, as shown by the dashed line in a . The egg chamber rotates within the surrounding basement membrane (illustration adapted from ref. 32 ). Full size image Although initially spherical, egg chambers lengthen along their anterior–posterior axes as they mature ( Fig. 1a ) [2] , [3] , [4] . This morphogenesis begins at stage five and depends on a precise organization of the basal epithelial surface, in which parallel arrays of actin bundles within the cells and fibril-like structures in the adjacent basement membrane align perpendicular to the elongation axis ( Fig. 1c ) [5] , [6] . This circumferential arrangement of structural molecules is thought to act as a ‘molecular corset’ that directionally biases egg chamber growth towards the poles, as mutations that disrupt this pattern lead to the production of round rather than elongated eggs [6] , [7] , [8] , [9] , [10] , [11] , [12] . Elongation also depends on an intriguing collective cellular motion, in which the entire egg chamber rotates perpendicular to the anterior–posterior axis within its surrounding basement membrane ( Fig. 1d ) [10] . The discovery that egg chamber elongation depends on rotation has led to two major challenges in understanding this system. The first is to determine the mechanisms underlying individual follicle cell motility. The second is to determine the relationship between the rotational motion and the morphogenesis itself. There is compelling evidence that rotation builds the polarized basement membrane associated with the molecular corset [10] . However, the relationship between rotation and the actin-based component of the corset, the basal actin bundles, remains unknown. The tissue-level organization of the basal actin bundles has been reported to fluctuate during the early stages of egg chamber development. The actin bundles first show a circumferential arrangement within the follicle cell precursors in the germarium [9] . However, this early tissue-level organization was reported to be lost on egg chamber formation, such that the basal actin bundles were still aligned within individual cells, but their global orientation was perturbed. The tissue-level alignment of the basal actin bundles was then thought to re-emerge at stage five, concurrent with the time that rotation and basement membrane polarization were reported to begin [9] , [10] . Recent work has shown that when rotation ends at stage nine, the actin bundles undergo oscillating, Myosin II-mediated contractions to produce a circumferentially constrictive force around the egg chamber to further elongate the tissue [13] . Here we show that egg chamber rotation is driven by lamellipodial protrusions at each follicle cell’s leading edge. We further show that rotation begins much earlier than previously reported, and that this motion is required for the tissue-level alignment of the basal actin bundles. By blocking rotation at discrete time points and employing a new quantitative method to characterize actin organization, we find that the actin-based component of the molecular corset is built in three steps. Global actin bundle alignment is first established among the follicle cell precursors in the germarium [9] . Contrary to previous reports, however, the tissue-level actin pattern is maintained by egg chamber rotation during stages one through five. Starting at stage six, rotation becomes dispensable for tissue-level actin bundle alignment. This change coincides with basement membrane polarization, which suggests that interactions between the basal actin bundles and the fibrillar matrix may stabilize the corset pattern. This work sheds light on the cellular mechanisms that drive egg chamber rotation and demonstrates how collective cell migration can be harnessed to build a tissue-level actin organization required for organ morphogenesis. Follicle cells have leading edge filopodia and lamellipodia To elucidate the cellular mechanisms underlying egg chamber rotation, we first investigated the composition of the actin cytoskeleton at the basal surface of the follicular epithelium. In addition to the parallel arrays of actin bundles, previous reports have identified a series of actin-based protrusions [14] , [15] . To determine whether the protrusions correspond to each follicle cell’s leading edge, we clonally expressed a fluorescently labelled actin-binding protein, Moesin ABD, and analysed egg chambers during stages six through eight. This labelling shows that actin-rich protrusions are uniformly restricted to one side of each cell ( Fig. 2a ). Furthermore, live imaging performed during the same stages reveals that membrane projections extend in the same direction as epithelial movement, indicating that they correspond to each migrating cell’s leading edge ( Fig. 2b and Supplementary Movie 1 ). 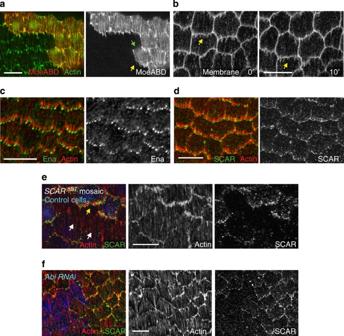Figure 2: Filopodia and lamellipodia form the leading edge of each migrating follicle cell. Laser-scanning confocal images were taken at the basal surface of stage seven and eight egg chambers. Scale bars, 10 μm. (a) The actin-binding domain of Moesin (MoeABD mCherry) was expressed in a clone of follicle cells (red) and the total F-actin population was labelled with phalloidin (green). Protrusions extend from only one side of each cell (yellow arrow) and not the other (green arrow). (b) Neuroglian (Nrg) and I’m not dead yet (Indy) GFP protein traps were used to visualize follicle cell membranes. Live imaging shows that membrane protrusions extend at the leading edge of the follicle cells. A single leading edge is indicated by the yellow arrow at 0 and 10 min. The arrows show that the protrusive activity and migration both occur in a downward direction. (c) Endogenous Ena localizes to the tips of filopodia. (d) Endogenous SCAR localizes more broadly within the leading edge protrusions, revealing the lamellipodia. (e) In aSCARΔ37mosaic egg chamber, the leading actin networks underlying the protrusions are absent in follicle cells lacking SCAR (white arrows). Control cells (blue) maintain SCAR localization with the leading edge protrusions (yellow arrow). (f) Clonal expression ofAbi RNAi(blue) also eliminates SCAR enrichment and protrusions at the leading edge. Figure 2: Filopodia and lamellipodia form the leading edge of each migrating follicle cell. Laser-scanning confocal images were taken at the basal surface of stage seven and eight egg chambers. Scale bars, 10 μm. ( a ) The actin-binding domain of Moesin (MoeABD mCherry) was expressed in a clone of follicle cells (red) and the total F-actin population was labelled with phalloidin (green). Protrusions extend from only one side of each cell (yellow arrow) and not the other (green arrow). ( b ) Neuroglian (Nrg) and I’m not dead yet (Indy) GFP protein traps were used to visualize follicle cell membranes. Live imaging shows that membrane protrusions extend at the leading edge of the follicle cells. A single leading edge is indicated by the yellow arrow at 0 and 10 min. The arrows show that the protrusive activity and migration both occur in a downward direction. ( c ) Endogenous Ena localizes to the tips of filopodia. ( d ) Endogenous SCAR localizes more broadly within the leading edge protrusions, revealing the lamellipodia. ( e ) In a SCAR Δ 37 mosaic egg chamber, the leading actin networks underlying the protrusions are absent in follicle cells lacking SCAR (white arrows). Control cells (blue) maintain SCAR localization with the leading edge protrusions (yellow arrow). ( f ) Clonal expression of Abi RNAi (blue) also eliminates SCAR enrichment and protrusions at the leading edge. Full size image Migrating cells typically have two types of actin-based protrusions at their leading edges that drive forward motility, filopodia and lamellipodia [16] , [17] . To determine whether both of these structures are present at the basal follicle cell surfaces, we stained for their characteristic markers. Enabled/VASP (Ena) is an actin-binding protein required for filopodia formation [18] . This protein localizes in a punctate pattern at the edge of the protrusions, consistent with localization to filopodial tips ( Fig. 2c ). The SCAR/Wave complex is an activator of the actin nucleator Arp2/3, which is required to produce the dynamic branched actin network of the lamellipodium [16] , [17] . SCAR localizes broadly across the leading edge of each follicle cell, consistent with localization to lamellipodial structures ( Fig. 2d ). Depletion of Ena changes protrusion morphology by eliminating the finger-like, filopodial actin structures ( Supplementary Figs 1a and 2a ). Under these conditions, SCAR still preferentially localizes to each follicle cell’s leading edge ( Supplementary Fig. 1b ). In contrast, loss of SCAR or depletion of the SCAR complex component Abelson interacting protein (Abi) eliminates all actin-based protrusions in a cell-autonomous manner, as well as the leading edge localization of Ena and SCAR ( Fig. 2e,f and Supplementary Fig. 1c ). Thus, the protrusive edge of each follicle cell contains both lamellipodia and filopodia. We next focused on the composition of the basal actin bundles and their relationship to the leading edge protrusions. We observed that non-muscle Myosin II and the focal adhesion component Paxillin localize along the length of the basal actin bundles while being largely excluded from the leading edge ( Supplementary Fig. 1d,e ). These results are consistent with previous reports suggesting the actin bundles are contractile stress fibres that mediate follicle cell attachment to the basement membrane [19] , [20] . Finally, we found that the protrusions can be separated spatially from the basal actin bundles within an individual cell. We have previously shown that tissue-level actin bundle alignment can be lost in a mosaic epithelium that contains a clone of cells lacking Misshapen kinase function [11] , [15] . Under these conditions, leading edge protrusions can extend orthogonally to the basal actin bundles in wild-type cells ( Supplementary Fig. 1f ). Moreover, complete loss of leading edge protrusions has no effect on the morphology or organization of the basal actin bundles ( Fig. 2e,f ). Altogether, these data indicate that the protrusive actin networks at the leading edge of each follicle cell are both compositionally and spatially distinct from the basal actin bundles. SCAR-dependent lamellipodia drive egg chamber rotation To determine the contribution of the leading edge actin networks to egg chamber rotation, we manipulated Ena and SCAR activity in the follicle cells. For these experiments, we used the traffic jam-Gal4 ( tj-Gal4 ) driver, which is expressed in both the follicle cell precursors and follicle cells at all developmental stages [21] . Depletion of Ena throughout the epithelium by RNA interference (RNAi) eliminates filopodia from the basal surface ( Supplementary Fig. 2a,b ) without disrupting rotation or egg chamber elongation ( Fig. 3a,b ). In contrast, depletion of Abi throughout the epithelium blocks egg chamber rotation ( Fig. 3a and Supplementary Movie 2 ). Similar to other perturbations that block rotation [10] , [15] , [22] , [23] , Abi depletion also disrupts basement membrane polarization, tissue-level actin bundle alignment and egg chamber elongation ( Fig. 3b–d ). When Abi is removed from a small clone of follicle cells, however, the cells that lack leading edge protrusions are carried along by their neighbours and rotation proceeds ( Supplementary Fig. 2c and Supplementary Movie 3 ). These findings show that Abi is required for egg chamber rotation, presumably due to its role in stimulating protrusive activity at each follicle cell’s leading edge. 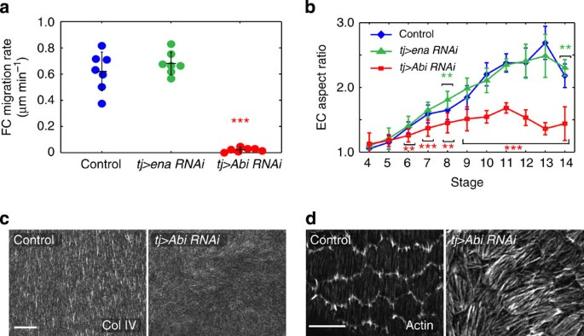Figure 3: SCAR-dependent lamellipodia promote egg chamber rotation. (a) Live imaging was used to determine the contributions of lamellipodia (Abi) and filopodia (Ena) to follicle cell (FC) migration. ExpressingAbi RNAiin all follicle cells throughout oogenesis with thetraffic jam-Gal4(tj-Gal4) driver blocks the rotation of stage seven–eight egg chambers, whereasena RNAihas no effect. Individual data points, mean±s.e.m.,t-test: ***P=1.7 × 10−7. (b)Abi RNAiegg chambers fail to elongate properly beginning at stage six, whereasena RNAidoes not disrupt elongation. The aspect ratio is the length of the egg chamber divided by its width. For stages 4–10n≥6, stages 11–13n≥3, stage 14n≥25 (exact n values are inSupplementary Table 2). Data represent mean±s.d.,t-test: **P<0.003, ***P<0.0008. (c) The basement membrane fails to become polarized when rotation is blocked by Abi depletion. Basement membrane structure is visualized using a GFP protein trap in the Collagen IV (Col IV) α2 chain, Viking (Vkg GFP). (d) Expression ofAbi RNAiwithtj-Gal4eliminates leading edge structures and disrupts the tissue-level alignment of the basal actin bundles. (c,d) Laser-scanning confocal images of stage seven-eight egg chambers. Scale bars, 10 μm. Figure 3: SCAR-dependent lamellipodia promote egg chamber rotation. ( a ) Live imaging was used to determine the contributions of lamellipodia (Abi) and filopodia (Ena) to follicle cell (FC) migration. Expressing Abi RNAi in all follicle cells throughout oogenesis with the traffic jam-Gal4 ( tj-Gal4 ) driver blocks the rotation of stage seven–eight egg chambers, whereas ena RNAi has no effect. Individual data points, mean±s.e.m., t -test: *** P =1.7 × 10 −7 . ( b ) Abi RNAi egg chambers fail to elongate properly beginning at stage six, whereas ena RNAi does not disrupt elongation. The aspect ratio is the length of the egg chamber divided by its width. For stages 4–10 n ≥6, stages 11–13 n ≥3, stage 14 n ≥25 (exact n values are in Supplementary Table 2 ). Data represent mean±s.d., t -test: ** P <0.003, *** P <0.0008. ( c ) The basement membrane fails to become polarized when rotation is blocked by Abi depletion. Basement membrane structure is visualized using a GFP protein trap in the Collagen IV (Col IV) α2 chain, Viking (Vkg GFP). ( d ) Expression of Abi RNAi with tj-Gal4 eliminates leading edge structures and disrupts the tissue-level alignment of the basal actin bundles. ( c , d ) Laser-scanning confocal images of stage seven-eight egg chambers. Scale bars, 10 μm. Full size image Egg chamber rotation begins at stage one Egg chamber rotation has been reported to begin at stage five [10] , [23] . However, we observed a polarized distribution of SCAR at the basal epithelial surface before this stage ( Fig. 4a ), which suggests that rotation may begin earlier than previously thought. Through long-term live imaging of entire ovarioles, we determined that egg chamber rotation begins at stage one and continues slowly through stage five before increasing in speed at stage six ( Fig. 4b,c , Supplementary Fig. 3a and Supplementary Movie 4 ). These data suggest that rotation occurs in two phases: an early slower phase and a later faster phase. Depletion of Abi from the follicle cells blocks the early as well as the late rotation ( Supplementary Fig. 3b ). To determine whether the early motion depends on other factors required for egg chamber rotation, we examined the atypical cadherin Fat2, which has been previously shown to be required for this motion at later stages [23] . Similar to depletion of Abi, loss of Fat2 function also disrupts egg chamber rotation during early stages ( Supplementary Fig. 3c and Supplementary Movie 5 ). Together, these data suggest that the two rotation phases depend on similar mechanisms driving follicle cell motility. 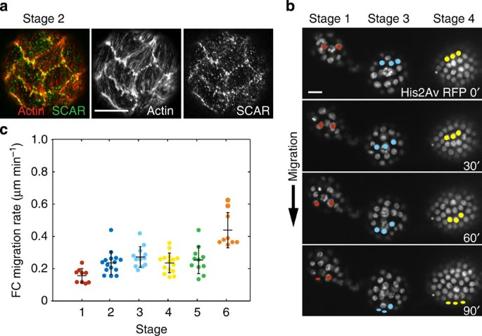Figure 4: Egg chamber rotation begins at stage one. (a) SCAR is enriched at one side of each follicle cell during early rotation stages. Scanning confocal image of the basal epithelial surface of a stage two egg chamber. (b) Stills from a time series of His2Av RFP-expressing egg chambers that show rotation occurring at stages one (0.10 μm min−1), three (0.34 μm min−1) and four (0.32 μm min−1). The coloured dots mark the same set of nuclei through each 30-min interval. Spinning disk confocal images. (c) Quantification of follicle cell (FC) migration rate. Each data point represents and individual egg chamber with mean±s.d. Scale bars, 10 μm. Figure 4: Egg chamber rotation begins at stage one. ( a ) SCAR is enriched at one side of each follicle cell during early rotation stages. Scanning confocal image of the basal epithelial surface of a stage two egg chamber. ( b ) Stills from a time series of His2Av RFP-expressing egg chambers that show rotation occurring at stages one (0.10 μm min −1 ), three (0.34 μm min −1 ) and four (0.32 μm min −1 ). The coloured dots mark the same set of nuclei through each 30-min interval. Spinning disk confocal images. ( c ) Quantification of follicle cell (FC) migration rate. Each data point represents and individual egg chamber with mean±s.d. Scale bars, 10 μm. Full size image Rotation maintains tissue-level actin bundle alignment As egg chamber rotation and the tissue-level alignment of the basal actin bundles were both thought to begin at stage five, it had been difficult to determine their order and dependence on one another. Given the finding that rotation actually begins at stage one, we can now investigate whether rotation plays a role in globally aligning the actin bundles. To this end, we developed a novel method to quantitatively assess basal actin bundle alignment from stages one through eight in rotating and non-rotating egg chambers. The epithelium was manually segmented into individual cells using cell membranes and cortical actin as markers, and each cell was then broken down into a series of small overlapping windows ( Fig. 5a and Methods). The orientation of the actin bundles in a given window was obtained by analysing the skew of its two-dimensional Fast Fourier Transform (2D FFT). Windows with aligned actin bundles produce asymmetrically skewed transforms, where the direction of skew is directly related to the orientation of the bundle ( Fig. 5b ) [24] . Iteratively performing this calculation yields a director field that represents a local measure of actin bundle orientation at a subcellular length scale ( Fig. 5c ). To determine the mean orientation of the actin bundles in a given cell, local directors ( Fig. 5c , green lines) were binned and averaged ( Fig. 5d , yellow lines). Finally, to determine the tissue-level polarity of the actin bundles, we defined a nematic order parameter ( S ) ( Fig. 5e ), which compares the relative orientation of cellular-level directors of all the cells within a given image ( Fig. 5d , yellow lines). The order parameter can vary from zero (random distribution of directors) to one (parallel directors), and was found to be independent of the size of the region analysed in the epithelial sheet ( Supplementary Fig. 4a,b and Supplementary Methods ). 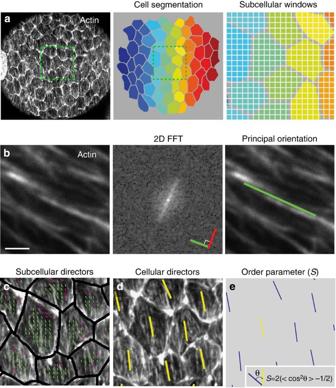Figure 5: Method for determining the global alignment of the basal bundles in a given epithelium. (a) Representative image of a stage five egg chamber where the actin is labelled with phalloidin (left panel). The pattern obtained by segmenting the epithelium into individual cells (centre panel). To analyse actin bundle alignment, individual cells are broken into subcellular windows of 6.74 μm2(right panel, windows are not shown to scale). (b) Representative image of the basal actin bundles in a subcellular window as defined ina. Scale bar, 2 μm. The 2D FFT of the actin image where the red line indicates the principal direction of the FFT, orthogonal to the orientation of actin bundles (centre panel, green line). Director indicating the local alignment of the actin image (left panel). (c) Magnification of the epithelial region within the green rectangle ina. Directors (green and magenta lines) indicate the local alignment of actin bundles within each cell. Directors deviating from the mean by more than an s.d. (magenta lines) were discarded (see Methods). (d) Director field showing the mean orientation (yellow lines) of the green directors within each cell shown inc. (e) The order parameter (S) is calculated by comparing the relative angle between all directors in an epithelium. Figure 5: Method for determining the global alignment of the basal bundles in a given epithelium. ( a ) Representative image of a stage five egg chamber where the actin is labelled with phalloidin (left panel). The pattern obtained by segmenting the epithelium into individual cells (centre panel). To analyse actin bundle alignment, individual cells are broken into subcellular windows of 6.74 μm 2 (right panel, windows are not shown to scale). ( b ) Representative image of the basal actin bundles in a subcellular window as defined in a . Scale bar, 2 μm. The 2D FFT of the actin image where the red line indicates the principal direction of the FFT, orthogonal to the orientation of actin bundles (centre panel, green line). Director indicating the local alignment of the actin image (left panel). ( c ) Magnification of the epithelial region within the green rectangle in a . Directors (green and magenta lines) indicate the local alignment of actin bundles within each cell. Directors deviating from the mean by more than an s.d. (magenta lines) were discarded (see Methods). ( d ) Director field showing the mean orientation (yellow lines) of the green directors within each cell shown in c . ( e ) The order parameter ( S ) is calculated by comparing the relative angle between all directors in an epithelium. Full size image Using this method we determined that the average tissue-level actin bundle alignment is high throughout stages one through eight, never falling below 70% of the maximum possible value ( Fig. 6a–c ). However, the average alignment does show a higher s.d. during stages one through four, which may account for previous reports that the basal actin bundles are not globally oriented during these stages [9] . Alignment then increases over time, reaching its peak at stages seven and eight. In contrast, when rotation is blocked with Abi RNAi or mutation of the fat2 gene, the global actin bundle pattern is indistinguishable from controls at stage one, but is then progressively lost starting at stage two ( Fig. 6a–c ). Consistent with these data, the actin bundles within the follicle cell precursors of the germarium are circumferentially aligned in all backgrounds ( Fig. 6d ). In both non-migratory conditions, actin bundle alignment is also preserved within individual cells at all developmental stages analysed ( Supplementary Fig. 4c ). These data indicate that rotation promotes actin bundle alignment on the tissue rather than cellular scale. 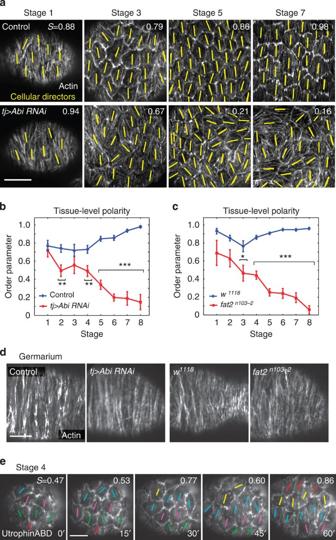Figure 6: Egg chamber rotation maintains the tissue-level alignment of the basal actin bundles. (a) Representative images of basal actin bundle alignment in control versusAbi RNAiepithelia at different stages with the corresponding order parameter value (S). Yellow lines represent the mean orientation of the basal actin bundles in each cell. Spinning disk confocal images. (b) Graph showing the average order parameters for control (blue line) versusAbi RNAi(red line) epithelia at stages one through eight. For stages 1–6n≥8, stage 7n≥5 and stage 8n≥4 (exactnvalues are inSupplementary Table 2). Data points represent mean±s.e.m.,t-test: **P<0.003, ***P<1.95 × 10−7. At-test compares the difference between control andAbi RNAiepithelia at each stage. (c) Graph showing the average order parameters for wild-type (blue) versusfat2n103-2(red) epithelia at stages one through eight. For stage 1n≥4, 2–5n≥7, 6n≥5, 7n≥8, 8n≥4 (exactnvalues are inSupplementary Table 2). Data points represent mean±s.e.m.,t-test: *P=0.012, ***P<5.96 × 10−7. At-test compares the difference between wild-type andfat2n103-2epithelia at each stage. (d) Basal actin bundles within the germarium are globally aligned in control,Abi RNAi, wild-type andfat2conditions. Spinning disk confocal images. (e) Stills from a 60-min near-total internal reflection fluorescence time series showing the basal actin bundles in a stage four egg chamber. The actin binding domain of Utrophin fused to GFP marks F-actin. The order parameter fluctuates, but there is a trend towards global actin bundle alignment. The coloured lines show the mean actin bundle orientation for each cell. Rows of cells sharing the same color can be followed through time to visualize the downward migration of the epithelium. Scale bars, 10 μm. Figure 6: Egg chamber rotation maintains the tissue-level alignment of the basal actin bundles. ( a ) Representative images of basal actin bundle alignment in control versus Abi RNAi epithelia at different stages with the corresponding order parameter value ( S ). Yellow lines represent the mean orientation of the basal actin bundles in each cell. Spinning disk confocal images. ( b ) Graph showing the average order parameters for control (blue line) versus Abi RNAi (red line) epithelia at stages one through eight. For stages 1–6 n ≥8, stage 7 n ≥5 and stage 8 n ≥4 (exact n values are in Supplementary Table 2 ). Data points represent mean±s.e.m., t -test: ** P <0.003, *** P <1.95 × 10 −7 . A t -test compares the difference between control and Abi RNAi epithelia at each stage. ( c ) Graph showing the average order parameters for wild-type (blue) versus fat2 n103-2 (red) epithelia at stages one through eight. For stage 1 n ≥4, 2–5 n ≥7, 6 n ≥5, 7 n ≥8, 8 n ≥4 (exact n values are in Supplementary Table 2 ). Data points represent mean±s.e.m., t -test: * P =0.012, *** P <5.96 × 10 −7 . A t -test compares the difference between wild-type and fat2 n103-2 epithelia at each stage. ( d ) Basal actin bundles within the germarium are globally aligned in control, Abi RNAi , wild-type and fat2 conditions. Spinning disk confocal images. ( e ) Stills from a 60-min near-total internal reflection fluorescence time series showing the basal actin bundles in a stage four egg chamber. The actin binding domain of Utrophin fused to GFP marks F-actin. The order parameter fluctuates, but there is a trend towards global actin bundle alignment. The coloured lines show the mean actin bundle orientation for each cell. Rows of cells sharing the same color can be followed through time to visualize the downward migration of the epithelium. Scale bars, 10 μm. Full size image To further characterize the dynamics of actin bundle orientation within individual migrating follicle cells, we performed live imaging of early rotation phase egg chambers. Consistent with the observation that the global actin alignment is more variable in young egg chambers, we found that the orientation of the actin bundle array within an individual cell can fluctuate as the epithelium migrates ( Fig. 6e and Supplementary Movie 6 ). Over time, the orientation is stabilized and the basal actin bundles are brought into alignment across the tissue. Altogether, these data are consistent with a model in which the tissue-level alignment of the basal actin bundles is established in the germarium, and that the global actin pattern is then maintained and reinforced by egg chamber rotation. Rotation becomes dispensable for global actin alignment One question that arose from the results above is whether rotation is continuously required to maintain tissue-level actin bundle alignment. To address this question, we developed methods to selectively block rotation at later stages. The mirror-Gal4 driver ( mirr-Gal4 ) [25] expresses weakly in the follicle cells at stages six and seven, and expresses highly at stage eight ( Supplementary Fig. 5a ). When Abi RNAi is expressed using mirr-Gal4 , egg chambers rotate and show proper basal actin bundle alignment at stage six. However, by stage eight, leading edge protrusions disappear ( Fig. 7a ) and 70% of the egg chambers have stopped rotating ( Supplementary Fig. 5b ). Significantly, the tissue-level alignment of the basal actin bundles is unaffected even though rotation has stopped prematurely. These data show that rotation becomes dispensable for maintaining the global actin pattern in stage-eight egg chambers. 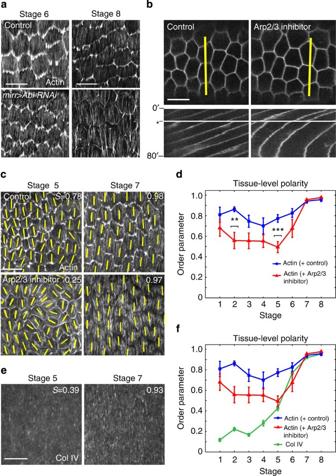Figure 7: Rotation is specifically required to maintain tissue-level actin alignment during early stages. (a) Late expression ofAbi RNAiusingmirror-Gal4(mirr-Gal4) does not affect the basal actin pattern at stage six but by stage eight, the leading edge actin network is eliminated without altering basal actin bundle alignment. One copy ofSCARwas also removed in this genetic background. Laser-scanning confocal images. (b) Kymographs of rotating egg chambers where the follicle cell membranes are marked with Indy GFP. The slopes of the indivdual lines indicate the rate at which the cell membranes are moving over time. After 20 min, the samples were treated with either with the Arp2/3 inhibitor CK-666 or the control molecule CK-689 (asterisk). The inhibitor stops follicle cell migration within 1 h.n=5 for each condition. Spinning disk confocal images. (c) Representative images of the basal actin bundle alignment after one hour of drug treatment during each of the given stages with the corresponding order parameter value (S). Yellow lines represent the mean orientation of the actin bundles in each cell. Spinning disk confocal images. (d) Graph showing the average order parameter for the basal actin bundles for stages one through eight after 1 h of drug treatment. The value is reduced in inhibitor-treated samples compared with controls only during early stages. During stages six to eight, the two values are indistinguishable. For stage 1n≥2, stages 2–3n≥6, stages 4–7n≥10, stage 8n≥4 (exactnvalues are inSupplementary Table 2). Data points represent mean±s.e.m. Thet-test compares the difference between the basal actin bundle order parameter in control and inhibitor-treated samples at each stage (**P=0.009, ***P=7.90 × 10−5). When stars are not shown, there was no statistically significant difference observed. (e) Representative images of basement membrane polarization (Col IV, Vkg GFP) with the corresponding order parameter value. Spinning disk confocal images. (f) Overlay of graphs fromdandSupplementary Fig. S5eshowing that the period when rotation becomes dispensable for the tissue-level actin alignment coincides with the period of highest basement membrane polarization. Scale bars, 10 μm. Figure 7: Rotation is specifically required to maintain tissue-level actin alignment during early stages. ( a ) Late expression of Abi RNAi using mirror-Gal4 ( mirr-Gal4 ) does not affect the basal actin pattern at stage six but by stage eight, the leading edge actin network is eliminated without altering basal actin bundle alignment. One copy of SCAR was also removed in this genetic background. Laser-scanning confocal images. ( b ) Kymographs of rotating egg chambers where the follicle cell membranes are marked with Indy GFP. The slopes of the indivdual lines indicate the rate at which the cell membranes are moving over time. After 20 min, the samples were treated with either with the Arp2/3 inhibitor CK-666 or the control molecule CK-689 (asterisk). The inhibitor stops follicle cell migration within 1 h. n =5 for each condition. Spinning disk confocal images. ( c ) Representative images of the basal actin bundle alignment after one hour of drug treatment during each of the given stages with the corresponding order parameter value ( S ). Yellow lines represent the mean orientation of the actin bundles in each cell. Spinning disk confocal images. ( d ) Graph showing the average order parameter for the basal actin bundles for stages one through eight after 1 h of drug treatment. The value is reduced in inhibitor-treated samples compared with controls only during early stages. During stages six to eight, the two values are indistinguishable. For stage 1 n ≥2, stages 2–3 n ≥6, stages 4–7 n ≥10, stage 8 n ≥4 (exact n values are in Supplementary Table 2 ). Data points represent mean±s.e.m. The t -test compares the difference between the basal actin bundle order parameter in control and inhibitor-treated samples at each stage (** P =0.009, *** P =7.90 × 10 −5 ). When stars are not shown, there was no statistically significant difference observed. ( e ) Representative images of basement membrane polarization (Col IV, Vkg GFP) with the corresponding order parameter value. Spinning disk confocal images. ( f ) Overlay of graphs from d and Supplementary Fig. S5e showing that the period when rotation becomes dispensable for the tissue-level actin alignment coincides with the period of highest basement membrane polarization. Scale bars, 10 μm. Full size image To determine precisely when rotation contributes to tissue-level actin alignment, we acutely blocked migration using the Arp2/3 inhibitor CK-666 (ref. 26 ). Egg chambers treated with the inhibitor stop rotating within an hour, whereas egg chambers treated with the control molecule CK-689 continue to rotate normally ( Fig. 7b and Supplementary Movie 7 ). Similar to late expression of Abi RNAi , stage-seven egg chambers treated with the inhibitor preserve their global actin bundle alignment in the absence of migration ( Supplementary Fig. 5c and Supplementary Movie 8 ). We treated egg chambers of all stages with the inhibitor or control molecule for 1 h and then immediately fixed them for analysis. Blocking rotation with the inhibitor causes the tissue-level actin alignment to drop below control levels for stages two through five. However, during stages six through eight the tissue-level actin pattern persists in the absence of migration ( Fig. 7c,d ). These data show that the early rotation phase is essential to maintain the tissue-level actin bundle alignment, but at later stages the pattern is preserved by an alternate mechanism. Previous work has shown that one of the functions of egg chamber rotation is to polarize the follicular basement membrane [10] . We hypothesize that this fibrillar matrix may preserve the tissue-level alignment of the basal actin bundles during stages six through eight by providing a stable source of polarizing information to the follicular epithelium. To investigate this possibility, we analysed the dynamics of basement membrane polarization through time and directly compared the results with the global actin alignment in rotating versus acutely blocked egg chambers. In agreement with previously published data, we find that basement membrane polarization increases through time, reaching its maximum at stages seven and eight ( Fig. 7e and Supplementary Fig. 5d,e ) [10] . When rotation is acutely blocked with the Arp2/3 inhibitor, any polarization that was already present in the matrix remains intact ( Supplementary Fig. 5f ). Importantly, there is a strong correlation between the period of maximal basement membrane polarization and the period when rotation becomes dispensable for maintaining the global actin bundle pattern ( Fig. 7f ). These data suggest that an interaction between the basal actin bundles and polarized basement membrane may maintain the tissue-level alignment of these structures at later developmental stages. Here we have shown that egg chambers begin rotating shortly after they emerge from the germarium and that this motion is driven by SCAR-dependent lamellipodia at each follicle cell’s leading edge. Thus, the well-studied mechanisms that underlie individual cell motility also promote the collective migration of the follicle cells that causes the egg chamber to rotate. There is growing evidence that coherent rotational motion may be an intrinsic property of epithelial tissues that adopt circular or spherical geometries [27] , [28] , [29] , [30] , [31] , [32] , [33] , [34] . This work highlights how epithelial rotation can be harnessed to organize a tissue for morphogenesis. It has been previously established that egg chamber rotation creates a system of polarized fibril-like structures in the follicular basement membrane required for egg chamber elongation [10] . Our data now show that rotation also promotes the tissue-level alignment of the second component of the molecular corset, the basal actin bundles. Based on our findings and those of others, we propose a three-step model for the formation of the molecular corset driving egg chamber elongation ( Fig. 8 ). First, the basal actin bundles become globally aligned within the follicle cell precursors in the germarium [9] . Second, this tissue-level actin pattern is inherited by a stage one egg chamber and is then maintained by the newly discovered early rotation phase. Third, rotation creates the fibrillar pattern in the basement membrane [10] , which then reinforces and stabilizes global actin bundle alignment through local cell–matrix interactions starting at stage six. In this way, epithelial rotation could provide a single mechanism to actively maintain, and then fix the actin-based component of the corset required for egg chamber elongation. 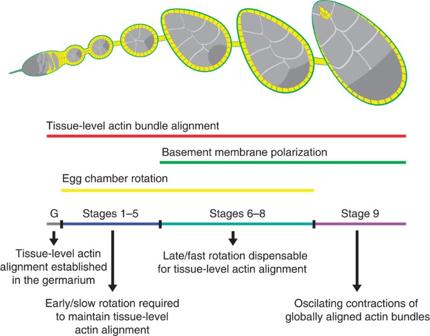Figure 8: Model for the formation of the actin-based component of the molecular corset for egg chamber elongation. Tissue-level alignment of the basal actin bundles is established in the germarium. Slow rotation occurs between stages one and five. This phase of rotation is required to maintain tissue-level actin bundle alignment. Fast rotation occurs between stages six and eight but is dispensable for the maintenance of the global actin pattern. This phase correlates with the polarization of the basement membrane, which may function to stabilize the actin pattern. Tissue-level polarization of the actin bundles and the basement membrane is maintained after migration stops at stage nine and the oscillating actin bundle contractions begin. Figure 8: Model for the formation of the actin-based component of the molecular corset for egg chamber elongation. Tissue-level alignment of the basal actin bundles is established in the germarium. Slow rotation occurs between stages one and five. This phase of rotation is required to maintain tissue-level actin bundle alignment. Fast rotation occurs between stages six and eight but is dispensable for the maintenance of the global actin pattern. This phase correlates with the polarization of the basement membrane, which may function to stabilize the actin pattern. Tissue-level polarization of the actin bundles and the basement membrane is maintained after migration stops at stage nine and the oscillating actin bundle contractions begin. Full size image Going forward, there are two major questions to address concerning the relationship between early rotation and tissue-level actin bundle alignment: Why is rotation required for this process, and what is the underlying mechanism? We hypothesize that early rotation transmits polarity information across the plane of the growing epithelium. From stages one to six, the number of follicle cells increases approximately tenfold [1] . As these cells migrate as a sheet, we envision that newly formed daughter cells can quickly establish a front–rear axis through positional cues from their neighbours. An individual follicle cell may then preferentially orient the polymerizing ends of its basal actin filaments towards the leading edge and the depolymerizing ends towards the trailing edge; however, the dynamics of the individual actin bundles remain to be investigated. Future work will also be required to determine how the actin bundles become organized into parallel arrays within each cell, as this phenomenon is not rotation dependent. Notably, it is not the lamellipodial actin networks themselve that orient the contractile actin bundles. We have shown that when an egg chamber contains a small clone of Abi RNAi follicle cells, rotation continues and the mutant cells are carried along. Under these conditions, the depleted cells lack leading edge protrusions but their basal actin bundles still show proper tissue-level alignment ( Fig. 2f ). Moreover, in wild-type cells, the leading edge actin networks can be oriented at a 90° angle from the basal actin bundles ( Supplementary Fig. 1f ). In classic planar cell polarity systems, the presence of a small mutant clone can produce a phenotype in which planar polarity is perturbed in and around the clone, but is normal elsewhere in the tissue [35] . In contrast, the tissue-level orientation of the basal actin bundles is an all-or-nothing process. This phenomenon was first noted for fat2 mosaic egg chambers [12] . When fat2 mutant cells make up <60% of the epithelium, tissue-level actin bundle alignment is normal; when mutant cells exceed 60%, actin bundle orientation is globally perturbed. This all-or-nothing relationship also holds true for epithelia that are mosaic for Abi function (this work) or Misshapen function [15] . The model that emerges is that the deciding factor between global actin bundle alignment and global perturbation is whether there are enough wild-type cells in the epithelium to allow bulk tissue movement (that is, rotation) to proceed. It will also be important to determine how tissue-level alignment of the basal actin bundles is maintained after stage five when rotation is no longer required. Several lines of evidence suggest that the fibrillar basement membrane matrix provides this stabilizing function. The basal actin bundles are known to interact with the basement membrane through integrin-based adhesions [7] , [13] , [19] . Moreover, we have shown that the peak polarity of the matrix correlates with the period when global actin bundle alignment is most coherent and when rotation becomes dispensable for this pattern. A continued stable interaction between the basal actin bundles and the polarized matrix may also provide the necessary foundation for the Myosin-mediated, oscillating contractions of the actin bundles that promote egg chamber elongation after rotation ceases [13] . Testing this hypothesis will ultimately require a better understanding of how basement membrane fibrils form. Other than blocking rotation before fibril formation, the only known method for eliminating these structures involves reducing matrix protein levels, which also affects rotation dynamics [10] . Whether it is the fibrillar matrix or some other polarized feature of the epithelium that preserves the actin bundle alignment, our results highlight how collective cell migration can be used to build a polarized, tissue-level actin network necessary for organ morphogenesis. Drosophila genetics Full genotypes for each experiment are provided in Supplementary Table 1 . For most experiments, crosses were raised at 25 °C and experimental females were aged on yeast for 1–3 days at the same temperature. Exceptions include His2AvRFP, which was kept and aged at room temperature, and SCAR Δ37 / mirr-Gal4; UAS-Abi-RNAi/+ along with the corresponding controls, which were aged at 29 °C. msn 102 mosaic egg chambers were produced using FRT80B with e22c-Gal4 driving FLP recombinase expression. SCAR Δ37 mosaic egg chambers were produced using FRT40A with GR1-Gal4 driving FLP recombinase expression. For flipout clones, UAS lines were crossed to flies containing the FLP recombinase under a heat shock promoter as well as the act5c»Gal4, UAS-GFP (or UAS-RFP ) flipout cassette. The heat shock was induced by incubating third instar larvae and pupae at 37 °C for 1 h with a 1-h recovery period at 25 °C followed by another hour at 37 °C for 3 × over 2 days. Females that eclosed during the heat shock process or the following day were placed on yeast with males overnight and dissected the next day. Most stocks were obtained from the Bloomington Stock Center with the following exceptions. vkg-GFP (CC00791), indy-GFP (CC00377) and Nrg-GFP (G00305) are from the Carnegie Protein Trap Library [36] . tj-Gal4 (104055) and UAS-Abi-RNAi are from the Drosophila Genetic Resource Center in Kyoto. UAS-ena-RNAi is from the Vienna Drosophila Resource Center . UAS-UtrophinABD::GFP is from T. Lecuit [37] , Sqh-Sqh::mCherry is from E. Wieschaus [38] and UAS-Pax::GFP is from D. Montell [13] . GR1-Gal4 , UAS-FLP was a generous gift from T. Schüpbach. UAS-MoeABD::mCherry was a generous gift from B. McCartney. Time-lapse image acquisition and microscopy One- to three-day-old females were aged on yeast with males for 1–3 days before dissection. Ovaries were dissected as described (see methods paper by Prasad et al . [39] ) in live imaging media. As young egg chambers are more prone to damage during the dissection process and damaged egg chambers do not rotate, all egg chambers were inspected for damage before and after imaging. When possible, 6 μM FM4–64 (Invitrogen) membrane dye was added to the live imaging media to highlight damaged tissue. ImageJ and Adobe Photoshop were used for image processing. For imaging performed on an upright scanning confocal microscope, ovarioles were transferred in live imaging media to an agar pad (live imaging media with 0.4% NuSieve GTG low-melt agarose) that was formed on a gas permeable membrane slide (Greiner Bio-One, discontinued product). Most of the live imaging media was removed from the pad and a coverslip was placed on top of the sample, stabilized with vacuum grease at each corner. The coverslip was then gently compressed onto the sample and halocarbon oil 27 (Sigma) was added around the coverslip to keep the media from evaporating. Egg chambers were imaged with × 40/1.3 numerical aperture (NA) EC Plan-NeoFluor oil-immersion objective on a laser-scanning confocal microscope (Zeiss LSM510) controlled by the LSM acquisition software. For near-total internal reflection fluorescence imaging [40] , [41] , [42] , ovarioles were transferred in live imaging media to a coverslip that was fused with melted parafilm to an aluminum slide with a 12-mm circular cut out. Twenty-micrometre polystyrene beads (Bangs Laboratories Inc.) were added to the media and a 16-mm 2 coverslip was placed on top of 4–5 ovarioles and 5–10 beads to compress the egg chambers against the bottom coverslip [41] . Egg chambers were imaged with a × 100/1.49 NA CFI Apo oil-immersion total internal reflection fluorescence objective (Nikon) using an Andor iXon3 897 EM-CCD camera on an inverted microscope (Ti-E; Nikon) controlled by Metamorph software (Molecular Devices). For imaging performed on an inverted spinning disk microscope, ovarioles were transferred into 37 °C live imaging media with 0.8% NuSieve GTG low-melt agarose on the aluminum slide. Ovarioles either sank in the media or were gently moved to the bottom with an eyelash tool before the media solidified at room temperature. The gas permeable membrane was placed on top of the slide to prevent evaporation. Egg chambers were imaged on an inverted microscope (Ti-E; Nikon) with a spinning disk confocal unit (CSUX; Yokogawa Electric Corporation) and an HQ2 camera (Roper Scientific) or a Rolera em-c 2 camera (Q imaging) using a × 60/1.2 NA Plan Apo water immersion objective (Nikon) or × 20/0.75 NA Plan Fluor multi-immersion objective (Nikon) controlled by Metamorph software. Immunohistochemistry Ovaries were dissected in S2 media warmed to room temperature and fixed in PBS+0.1% Triton+4% EM-grade formaldehyde (Polysciences). For actin staining only, ovaries were washed 3 × in PBS+0.1% Triton (PBT), then egg chambers were disrupted from the muscle sheath by gentle pipetting. Staining was performed with rhodamine phalloidin (1:200, Sigma), AlexaFluor-488 Phalloidin (1:200, Invitrogen) or AlexaFluor-647 Phalloidin (1:75, Invitrogen) for 15 min in PBT at room temperature while rocking. Egg chambers were then washed 3 × in PBT and mounted in SlowFade Antifade (Invitrogen). Egg chambers stained with primary antibodies were incubated overnight at 4 °C with rocking in PBT+0.1% BSA+Phalloidin. Egg chambers were incubated in AlexaFluor-488- or 555-conjugated secondary antibodies (1:200, Invitrogen) in PBT+0.1% BSA+Phalloidin for 3 h at room temperature with rocking. The following primary antibodies were used: anti-Ena (1:200 concentrate, DSHB), anti-SCAR (1:300) [43] and anti-SCAR (1:200 concentrate, DSHB) [44] . For SCAR staining, primary and secondary incubations along with all washes following the primary incubation, PBT3 (PBS+0.3% Triton) was used instead of PBT. Fixed egg chambers were imaged with a laser-scanning confocal or a spinning disk confocal (described above). Image J and Adobe Photoshop were used for image processing. Drug treatment To show that egg chamber rotation can be acutely disrupted with a pharmacological treatment, ovaries were dissected as stated above in live imaging media with 2.5% dimethyl sulphoxide (DMSO). Ovarioles were transferred in the live imaging media to the aluminum slide and imaged on an inverted spinning disk microscope. After 20 min, the imaged ovarioles were quickly washed 3 × in live imaging media with 2.5% DMSO and 250 μM of the Arp2/3 inhibitor (CK-666, Millipore) [26] or control molecule (CK-689, Millipore), and imaged in the third wash for an additional hour. To visualize the actin cytoskeleton in drug-treated egg chambers live, UtrophinABD::GFP-expressing ovarioles were dissected in live imaging media with the inhibitor and imaged on the laser-scanning confocal microscope as described above. For fixed images, three females were dissected per experiment in live imaging media with 2.5% DMSO and 250 μM of the inhibitor or control molecule. Approximately 20 ovarioles were incubated for 1 h then fixed and stained with Phalloidin as described above. Quantification of egg chamber rotation rate Rotation speed was measured from time-lapse images of egg chambers expressing His2AvRFP or a membrane-targeted green fluorescent protein (GFP). A line was drawn over a row of follicle cells in the direction of migration to generate kymographs. Migration rates were obtained from the slope of the lines in the kymograph. All analyses were performed using Metamorph software (Molecular Devices). Quantification of cell-level actin bundle alignment Actin bundle orientation was calculated using fixed samples where F-actin was labelled with phalloidin. A local director representing actin alignment was determined as follows. First, each image was broken down into a series of 2.6 μm by 2.6 μm overlapping windows. A symmetric Gaussian filter was applied to each window to minimize edge effects and the 2D FFT of the filtered window was calculated. Windows with oriented actin bundles resulted in asymmetrically skewed transforms, where the direction of skew is directly related to the orientation of the actin bundle. Windows with no predominant orientation yielded a uniform transform. The principle direction of the skewed transform was determined by calculating the angle of the axis for the least second moment of the transform. The average orientation of the actin in real space (that is, image window) is orthogonal to the principle direction of the skewed transform in frequency space (the 2D FFT). To determine the direction of alignment at the cellular scale, we averaged the directors within each cell. Only directors within 1 s.d. of the mean were included in this average ( Fig. 5c , green lines), as outliers were often the product of edge effects in the analysis ( Fig. 5c , magenta lines). All calculations were performed using custom-written routines in MATLAB. Quantification of tissue-level actin bundle alignment To assess the tissue-level alignment of the basal actin bundles, we calculated an order parameter, S , for each egg chamber by considering the directors of all the cells visible in an image, as determined above. We defined S as: Where θ ij is the angle between the directors of cells i and j . The average was performed over all unique cell pair combinations in an image. S ranges from zero (randomly oriented directors) to one (parallel directors). As cells visible in a fixed image corresponded only to a fraction of the entire epithelium, we tested whether measuring local order (a limited number of cells) was representative of global polarity patterns (the entire egg chamber). We first binned each egg chamber into regions that included an increasing number of adjacent/neighbouring cells. The size of the bin varied from two (adjacent cells only) up to n -connected cells, where n was the maximum distance (in cells) between two visible cells in an image. The order parameter S was calculated for each bin and averaged over regions of the same connectivity in egg chambers of the same developmental stage. We observed no dependence of the average order parameter on the size of the region analysed ( Supplementary Fig. 4 ). Thus, our local measurements can be taken as representative of global actin bundle organization in the egg chamber. Quantification of Collagen IV organization Collagen IV orientation was calculated from fixed egg chambers expressing Vkg-GFP. Each image was broken down into windows (50 × 50 pixels per 20.06 μm 2 ) that overlapped by 2.23 μm. A director was obtained for each window following the same procedure described for the actin bundles. The order parameter, S , of the director field obtained was then calculated to quantify the orientation of fibril-like structures in the basement membrane. Statistical analysis and data reproducibility For the representative images shown in Figs 2 , 3c,d , 4a , 6d and 7a and Supplementary Figs 1, 2 and 5a , consistent results were obtained from at least two independent experiments. For each experiment, at least five female flies were dissected and multiple egg chambers were analysed. There were no limitations on data reproducibility. For the aspect ratio graph shown in Fig. 3b , the data were obtained from two independent experiments. For each experiment, ten female flies were dissected and multiple egg chambers were analysed at each developmental stage. Exact n values are in Supplementary Table 2 . For the measurements of basal actin bundle alignment and basement membrane polarization shown in Figs 5 , 6 and 7c–f , and Supplementary Figs 4 and 5d–f , the data were obtained from at least four independent experiments. For every experiment, at least five female flies were dissected and multiple egg chambers were analysed at each stage. Exact n values are in Supplementary Tables 2 and 3 . Live imaging experiments were performed at least two independent times with consistent results. For each experiment, three female flies were dissected. For all experiments, damaged egg chambers were excluded from the analysis. The experiments were not randomized. Rotation rates, basal actin bundle alignment and basement membrane polarization quantifications were performed without knowledge of egg chamber stage. One researcher recorded the stage and a second researcher performed the quantitative analysis blind. Blinding was not performed on other experiments. No statistical method was used to predetermine sample size. The sample sizes for each experiment are either shown as individual data points on the graph itself or are detailed in Supplementary Tables 2 and 3 . A Student’s t -test was used to determine whether data from two experimental conditions were significantly different. This test is appropriate, because all data obtained follow an approximately normal distribution, as determined by the three-sigma rule test. Differences between experimental and control conditions were large in all cases and the variability within a single experimental condition was low. How to cite this article: Cetera, M. et al . Epithelial rotation promotes the global alignment of contractile actin bundles during Drosophila egg chamber elongation. Nat. Commun. 5:5511 doi: 10.1038/ncomms6511 (2014).